Epigenetic diversity increases the productivity and stability of plant populations Biological diversity within species can be an important driver of population and ecosystem functioning. Until now, such within-species diversity effects have been attributed to underlying variation in DNA sequence. However, within-species differences, and thus potentially functional biodiversity, can also be created by epigenetic variation. Here, we show that epigenetic diversity increases the productivity and stability of plant populations. Epigenetically diverse populations of Arabidopsis thaliana produce up to 40% more biomass than epigenetically uniform populations. The positive epigenetic diversity effects are strongest when populations are grown together with competitors and infected with pathogens, and they seem to be partly driven by complementarity among epigenotypes. Our study has two implications: first, we may need to re-evaluate previous within-species diversity studies where some effects could reflect epigenetic diversity; second, we need to incorporate epigenetics into basic ecological research, by quantifying natural epigenetic diversity and testing for its ecological consequences across many different species. Humans depend on natural ecosystems to provide them with food and many other goods and services [1] . We now know that the biological diversity of these ecosystems is one of the key determinants of their functioning, which means that biodiversity loss may threaten the ecosystem processes on which we depend [2] , [3] , [4] , [5] . Although most observational or experimental functional biodiversity research has been conducted at the level of species diversity, there is increasing evidence that positive biodiversity–ecosystem functioning relationships also exist at the intraspecific level. Populations or communities composed of multiple genotypes of the same species are often found to be more productive, more resistant to natural enemies or invaders or more stable under stressful conditions than populations or communities that lack such intraspecific diversity [6] , [7] , [8] , [9] . So far, only DNA sequence variation has been considered capable of generating heritable functional differences between individuals, and therefore such effects of intraspecific diversity have been attributed to DNA sequence variation. However, recent evidence suggests that, even in the absence of DNA sequence variation, within-species variation in functional traits can be created by epigenetic variation [10] , [11] , [12] , [13] . Epigenetic modifications of the genome, such as DNA methylation or various histone modifications—which influence gene expression and thus, ultimately, the phenotypes of organisms—can vary across individuals or populations of the same species, and this variation can be heritable [14] , [15] . Only recently, ecologists and evolutionary biologists have recognized the potential relevance of epigenetic variation for their fields and begun to study it in an ecological-evolutionary context [16] , [17] . Results of these studies indicate that epigenetic variation is ubiquitous within and among natural plant populations [18] , [19] , [20] , [21] , [22] , and that epigenetic differences can be independent from DNA sequence variation [10] , [23] , [24] (although rigorous demonstrations of true independence are difficult and still scarce). Moreover, there is increasing evidence that epigenetic variation alone can create heritable variation in ecologically important traits such as the growth, phenology and herbivore defence of plants [11] , [12] , [25] , as well as in phenotypic plasticity, niche width and habitat differentiation [13] , [21] , [26] , [27] . If epigenetic variation can create heritable variation in functional traits, then epigenetic diversity could, in principle, have positive effects, similar to those of DNA sequence diversity, on the functioning of populations and ecosystems. To test this hypothesis, we conducted a greenhouse experiment ( Fig. 1 ) with plant populations differing in epigenetic diversity. We achieved this by working with epigenetic recombinant inbred lines (epiRILs) of Arabidopsis thaliana , lines that were derived from two parents with near identical genome sequence but highly contrasted DNA methylation profiles [25] . Previous research has shown that these epiRILs are highly variable in DNA methylation and represent a mosaic of their parents’ epigenomes, and that a large fraction of the DNA methylation differences among epiRILs are stably inherited for many generations [28] . Starting from a pool of 20 epiRILs, we created monocultures of each epiRIL, as well as populations composed of 2, 4 or 16 epiRILs, respectively, and we subjected these populations to a factorial combination of pathogen attack and weed competition. Our study shows that epigenetic diversity strongly increases the productivity of Arabidopsis populations, particularly in the presence of competitors and pathogens, and that epigenetically diverse populations are better able to suppress competitors. We conclude that epigenetic diversity can have similar functional consequences as other levels of diversity, and that it may represent an overlooked level of natural biodiversity that needs to be incorporated in basic ecological research. 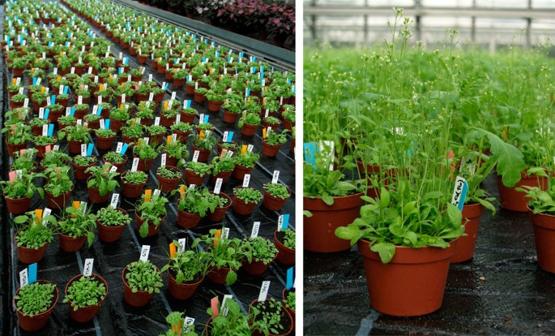Figure 1:ExperimentalArabidopsis thalianapopulations of different epigenetic diversity growing with or without weedy competitors.  Figure 1: Experimental Arabidopsis thaliana populations of different epigenetic diversity growing with or without weedy competitors. Full size image Epigenetic diversity effects Epigenetic diversity had a significant positive effect on the total biomass of Arabidopsis populations, and there were significant negative effects of both competition and pathogens on total biomass ( Table 1 ). On average, population composed of 16 epigenotypes achieved a 23% higher biomass than epigenetic monocultures. The effect was strongest in the presence of competitors and pathogens, where biomass production even increased by 44%. A similar diversity effect was found when we analysed plant density instead of total biomass ( Table 1 ). At the time of harvesting, rosette densities were 16% higher in the 16-epigenotype mixtures than in the monocultures, which suggests that part of the observed diversity–productivity relationships were mediated by changes in plant densities, a result also found in biodiversity experiments, which manipulated plant species diversity [29] . 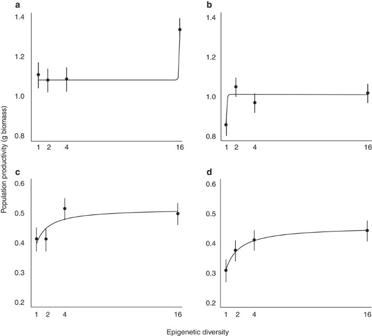Figure 2: Relationships between epigenetic diversity and productivity in each experimental treatment. Arabidopsis thalianapopulations composed of 1, 2, 4 or 16 different epigenetic recombinant inbred lines were grown under control conditions (a), infected with the pathogenPseudomonas syringae(b), grown in competition with two annual weeds (c) or subjected to both competition and pathogen infection (d). The data shown are average total population biomasses (± standard errors), based on 20 monoculture averages and 24 replicate populations per each other diversity level in each treatment, and the fitted lines represent the best fit models from a series of contrasts as well as linear and non-linear regression models. There was no effect of Arabidopsis epigenetic diversity on the biomass of its competitors, but we found a significant or marginally significant effect of epigenetic diversity on the phenology and reproductive output of the dominant competitor Senecio vulgaris ( Table 2 ), which flowered later and was less fecund in epigenetically diverse Arabidopsis populations. Thus, epigenetic diversity increased not only the productivity of the Arabidopsis populations but also their ability to suppress weedy competitors. Table 1 Effects of epigenetic diversity as well as pathogens and interspecific competitors on the productivity and density of A. thaliana populations. Full size table Table 2 Effects of Arabidopsis population epigenetic diversity and pathogens on the performance of the competitor species Senecio vulgaris. Full size table Shape of the diversity–productivity relationship Having established an effect of epigenetic diversity on population productivity, we tested for the specific shape of the diversity–productivity relationship. 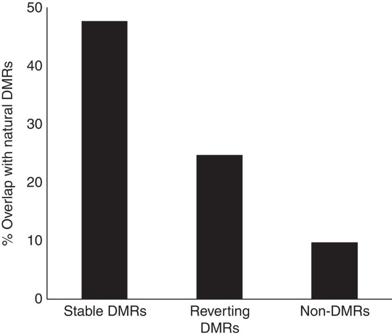Figure 3: Overlap of epigenetic polymorphisms between epiRILs and naturalArabidopsisaccessions. A total of 867 stable and 1,744 reverting differentially methylated regions (DMRs) as well as 1,333 regions equally methylated (non-DMRs) between the wild-type andddm1parents of the epiRIL population were compared with the 13,485 natural C-DMRs identified by Schmitzet al.22in 152 natural accessions ofArabidopsis thaliana. To explore this, we fitted a series of linear and non-linear models ( Table 3 ). As relationships tended to vary among treatments ( Table 1 ; marginally significant three-way interaction between epigenetic diversity, competition and pathogens), we analysed diversity–productivity relationships separately for each of the four treatment combinations. In all four cases, there was a significant relationship between epigenetic diversity and total Arabidopsis biomass ( Fig. 2 ), but the shapes of the relationships differed among treatments. In the control treatment, the best fit model represented diversity as the contrast between the 16-epiRIL diversity and all other diversity levels ( Fig. 2a ), which suggests that under these conditions only the highest level of epigenetic diversity increased productivity. In the pathogen-only treatment, diversity was best modelled as the contrast between monocultures and all other diversity levels ( Fig. 2b ), implying that in the presence of pathogens any level of epigenetic diversity had a positive effect on productivity. Finally, in the two competition treatments (with or without pathogens), the best fit models were Michaelis–Menten models ( Fig. 2c,d ), indicating saturating epigenetic diversity-productivity relationships and therefore some degree of redundancy between epigenotypes. Table 3 Results of model selection exploring the shapes of epigenetic diversity-productivity relationships. Full size table Figure 2: Relationships between epigenetic diversity and productivity in each experimental treatment. Arabidopsis thaliana populations composed of 1, 2, 4 or 16 different epigenetic recombinant inbred lines were grown under control conditions ( a ), infected with the pathogen Pseudomonas syringae ( b ), grown in competition with two annual weeds ( c ) or subjected to both competition and pathogen infection ( d ). The data shown are average total population biomasses (± standard errors), based on 20 monoculture averages and 24 replicate populations per each other diversity level in each treatment, and the fitted lines represent the best fit models from a series of contrasts as well as linear and non-linear regression models. Full size image Two mechanisms could have driven the diversity–productivity effects observed in our experiment: the higher likelihood of including a highly productive epigenotype in a diverse mixture (selection effect) or niche complementarity among different epigenotypes. Our experiment was not designed to disentangle the contributions of these two mechanisms [30] , [31] . This would have required harvesting and measuring individual seedlings of known epigenotypic identity, which would have been possible only with controlled, evenly spaced planting of seedlings with a much less realistic population structure. Nonetheless, we found that in 61 out of 288 cases the total biomass of a multi-epigenotype population exceeded the monoculture biomass of its most productive constituent epigenotype. As such transgressive overyielding is impossible without complementarity [31] , this strongly suggests that at least part of the observed diversity effects are due to niche complementarity among different epigenotypes. The net biodiversity effects observed in our study are substantial. In the control, pathogen-only and competition-only treatments, epigenetic diversity generally increased population productivity by around 20%, and in the competition plus pathogen treatment, productivity was even increased by 44% at the highest level of epigenetic diversity. These effect sizes are close to those found in a review of 44 species diversity experiments where species mixtures produced on average 72% more biomass than monocultures [31] . It is intriguing that, similarly as in other diversity studies [32] , the benefit of increased epigenetic diversity was greatest under the most realistic environmental conditions where both pathogens and competitors were present. The results of our study are comparable to previous species or within-species diversity experiments not only in terms of effect sizes but also in terms of the shape of the diversity–productivity relationships and the underlying mechanisms. We found that epigenetic diversity–productivity relationships were generally non-linear and tended to be saturating, which indicates that some functional redundancy exists among different epigenotypes. Moreover, the observed transgressive overyielding indicates that functional complementarity must play a role in the diversity effects. Both results are generally consistent with evidence from species diversity experiments [2] , [3] , [4] , [31] . Our study demonstrates that extensive variation in DNA methylation among nearly isogenic lines can in principle create functional diversity with similar general properties and positive effects on population and ecosystem processes as the functional diversity observed among different genotypes and species in nature [2] , [3] , [4] , [5] , [6] , [7] , [8] , [9] . One conclusion from our study is therefore that we may need to re-evaluate the results of many previous within-species diversity studies where diversity gradients were created by mixing plant material from different maternal lines or populations. With ubiquitous epigenetic variation in natural populations [18] , [19] , [20] , [21] , [22] , such mixtures may have been equally diverse at the epigenetic level, and therefore the observed ecological effects could have been caused by DNA sequence diversity, epigenetic diversity or both. The second, more general conclusion is that epigenetic diversity could potentially be highly relevant for basic ecological research. However, to understand its true relevance, we need to make the step from proof-of-principle to more realistic studies. In the epiRIL study system, levels of epigenetic diversity, and their effect sizes, may be at the upper limit of what is possible. Moreover, most natural populations will also exhibit DNA sequence diversity, which may or may not interact with epigenetic diversity in determining population productivity and stability. Thus, while our study provides strong proof-of-principle that epigenetic diversity alone can have significant ecological consequences, it remains difficult to predict effect sizes of epigenetic diversity, and its relative importance compared with genetic diversity, in natural populations. Therefore, the important next steps are to survey epigenetic diversity across many different species in wild populations, examine to what degree epigenetic diversity is independent from or interacts with genotypic diversity and test for the environmental correlates and ecological consequences of epigenetic diversity both experimentally and in the field. Plant material The epigenetic recombinant inbred lines (epiRILs) used in our study were derived from a cross of the hypomethylation mutant Col-ddm1 of Arabidopsis thaliana , which shows a 70% reduction of overall DNA methylation, with its wild type. After a backcross of the F1 with the wild type, inbred lines were established from F2 plants homozygous at DDM1 , which were thus nearly identical in DNA sequence, but, through recombination, differed greatly in their patterns of DNA methylation. Using stringent criteria, 2611 differentially methylated regions (DMRs) could be identified between the two parental lines, of which approximately one-third were stably inherited for at least eight generations [28] . Recent data show that these DMRs are even stable for over 16 generations in the epiRIL population ( Table 4 ). The epiRILs also show strong heritable differentiation in phenotype [11] , [12] , [13] , [25] , and it is highly likely that these phenotypic differences are the result of DNA methylation differences. Although DNA sequence differences exist in epiRILs (few leftover SNPs or changes in transposable elements that were inherited from the DDM1 parent or occurred during inbreeding), ongoing whole-genome resequencing indicates that differences in DNA sequence among epiRILs are several orders of magnitude smaller than differences in DNA methylation. Most importantly, ~50% of the stable DMRs present in the epiRIL population overlap with DMRs identified among Arabidopsis natural populations ( Fig. 3 ). More detailed descriptions of the epiRILs can be found elsewhere [25] , [28] . For our experiment, we selected a pool of 20 epiRILs of the F8 generation that represented the full range of phenotypic variation—based on a multivariate analysis of several growth, fitness and phenology traits—observed in a previous screening of 135 epiRILs [13] . Table 4 Stability of DNA methylation polymorphisms in epiRILs. Full size table Figure 3: Overlap of epigenetic polymorphisms between epiRILs and natural Arabidopsis accessions. A total of 867 stable and 1,744 reverting differentially methylated regions (DMRs) as well as 1,333 regions equally methylated (non-DMRs) between the wild-type and ddm1 parents of the epiRIL population were compared with the 13,485 natural C-DMRs identified by Schmitz et al. [22] in 152 natural accessions of Arabidopsis thaliana . Full size image Seeds of the two competitor species Poa annua and Senecio vulgaris were bought from a regional supplier of wild-collected seeds (Rieger-Hofmann GmbH, Blaufelden-Raboldshausen, Germany). Experimental design We established a total of 608 experimental populations, with monocultures replicated four times, and each other diversity level replicated 24 times, in each treatment. Each population was established by planting 48 Arabidopsis seeds, with all epiRILs at equal abundance, into 8-cm pots filled with a commercial seedling substrate (Klasmann-Deilmann GmbH, Geste, Germany). The seeds were spread randomly on the soil surface, which created dense populations with a realistic population structure. In total, we planted 29,184 seeds of A. thaliana , which resulted in 13,372 established plants at the time of harvest. For the multi-epigenotype populations, lines were selected randomly, with the condition that each individual mixture was unique and all 20 epiRILs were equally represented across populations within each treatment combination. In the competition treatment, we additionally planted 10 seeds of Poa annua and 10 seeds of Senecio vulgaris . In the pathogen treatment, we sprayed populations six times with the bacterial pathogen Pseudomonas syringae pv. tomato DC3000 at a concentration of 108 bacteria per cm 3 . The experiment was set up in early July 2011 in a greenhouse in Bern, Switzerland ( Fig. 1 ). The pots were watered regularly, and we twice added liquid fertilizer (N-P-K 18-12-18) at a concentration of 500 p.p.m. to the irrigation water. After six weeks, we harvested all aboveground biomass, counted the final number of Arabidopsis rosettes in each pot and determined the total dry weight of Arabidopsis . In the competition treatment, we also recorded the time to first flowering of Senecio , counted the numbers of Senecio flower heads and determined the total dry weight of Poa and Senecio . Statistical analyses Effects of epigenetic diversity on Arabidopsis rosette density and total population biomass were analysed with linear models that included the effects of epigenetic diversity (as a continuous variable), competition and pathogens, and all possible interactions between these variables ( Table 1 ). Epigenetic diversity effects on competitor biomasses as well as on Senecio phenology and fecundity were analysed with linear models that tested the effects of epigenetic diversity, pathogens and their interaction ( Table 2 ). In all analyses, we averaged monoculture biomasses across the four replicates. In addition to testing for overall effects of epigenetic diversity, we also explored the specific shape of the relationship between epigenetic diversity and Arabidopsis biomass. The shape of a diversity-function relationship has important implications both for the mechanisms underlying diversity effects and the consequences of diversity loss for functioning [33] . We therefore fitted a series of linear and non-linear models to the biomass data ( Table 3 ), similar to those used in other analyses [33] , [34] : a linear model, which implies equal functional effects and no redundancy among epigenotypes, two saturating models (Michaelis–Menten and asymptotic exponential), which would suggest some redundancy, a quadratic model, which would indicate an optimum level of epigenetic diversity and an exponential model, which would imply strong positive interactions among epiRILs and rapid loss of function if diversity is reduced. We also modelled diversity as a categorical variable, which would suggest differences between diversity levels but no clear increase in function with increasing diversity, and in addition we fitted two contrasts, to determine if the diversity effect was due to a particular diversity level differing from all the others: monocultures versus all other diversity levels and the highest diversity level (16 epiRILs) versus all other levels. We used AICc (AIC corrected for small sample sizes) to select the best fitting models within each treatment combination. We also calculated AICc weights for each model, which calculate the degree of support for a particular model relative to the others in the set. How to cite this article: Latzel, V. et al. Epigenetic diversity increases the productivity and stability of plant populations. Nat. Commun. 4:2875 doi: 10.1038/ncomms3875 (2013).